Trunk cleavage is essential forDrosophilaterminal patterning and can occur independently of Torso-like Terminal patterning in Drosophila is governed by a localized interaction between the Torso kinase (Tor) and its ligand Trunk (Trk). Currently, it is proposed that Trk must be cleaved in order to bind Tor, and that these proteolytic events are controlled by secretion of Torso-like (Tsl) only at the embryo poles. However, controversy surrounds these ideas since neither cleaved Trk nor a protease that functions in terminal patterning have been identified. Here we show that Trk is cleaved multiple times in vivo and that these proteolytic events are essential for its function. Unexpectedly, however, the Trk cleavage patterns we observe are unaltered in tsl -null mutants. One explanation for these data is that the influence of Tsl on localized Trk cleavage at the embryo poles is subtle and cannot be readily detected. Alternatively, we favour a scenario where Tsl functions post proteolytic processing of Trk to control localized terminal patterning. Patterning of the Drosophila embryo depends on spatial cues provided by maternal gene products and has served as a model paradigm for studying the localized activation of important developmental signalling pathways such as Toll and receptor tyrosine kinase signalling. In Drosophila , terminal patterning is achieved by localized activation of the Torso (Tor) receptor tyrosine kinase. The proposed ligand for Tor is Trunk (Trk), a protein that is most similar to the Noggin-like branch of the cysteine-knot superfamily [1] , [2] . Other notable cysteine knot-like family members in Drosophila include Spätzle (Spz), the growth factor that binds the Toll receptor, thus initiating dorsoventral patterning [3] , [4] . In this system, the Spz ligand is generated through the actions of a complex extracellular proteolytic cascade [4] . Given that Trk has the same cysteine knot-like fold as Spz [5] , it has been previously suggested that Trk might be cleaved in order to bind and activate the Tor receptor [5] . In support of these ideas, Casali and Casanova [6] used the Easter protein signal peptide to express shortened Trk variants (lacking either 76 or 127 amino acids in the amino terminus) in the extracellular region between the oocyte cytoplasmic membrane and vitelline membrane (the perivitelline (PV) space). These constructs were able to ubiquitously activate Tor signalling and bypass other known maternal factors, albeit inefficiently. In addition to suggesting a requirement for Trk proteolytic processing, these studies also strongly implicate Trk as the Tor ligand in terminal patterning. Further, it is notable that a second Tor ligand, prothoracicotropic hormone, lacks a Trk-like N-terminal region [1] and can constitutively activate Tor in the absence of other factors [7] . Despite these findings, a major question in terminal patterning remains unsolved—how is Tor signalling localized to the embryonic poles? The homogeneous distribution of tor messenger RNA in embryos [8] , in addition to several lines of genetic evidence [9] , [10] , [11] suggests that Tor is present ubiquitously on the embryo plasma membrane. Similarly, Trk is also produced in the oocyte and, while its trafficking remains to be understood, it is suggested that it is secreted into the PV space [5] , [11] . Currently, the only known localized factor in the terminal patterning pathway is Torso-like (Tsl)—a membrane attack complex/perforin-like (MACPF) protein that is secreted from specialized follicle cells at the anterior and posterior ends of the oocyte [9] , [11] , [12] . Homozygous tsl -mutant females produce embryos that lack all terminal structures, characteristic of the terminal-class genes. Importantly, however, ectopic expression of Tsl from all follicle cells produces ubiquitous Tor signalling, resulting in expanded terminal regions at the expense of the central segments [10] , [12] . Given its specific localization at the poles, and the likely requirement for Trk cleavage, it has been proposed that Tsl permits a protease to cleave Trk into its active form only at the embryo poles [6] . However, in contrast to the dorsoventral patterning system, where a major cascade of proteases and regulatory serpins are known and characterized [14] , to date no protease required for terminal patterning has been found, nor has a cleaved Trk species been identified. Here we provide direct evidence of Trk proteolytic processing in protein extracts from early embryos, finding that it is cleaved multiple times. We also show that this cleavage is necessary for its function in the activation of Tor. Finally, we test the long-standing idea that Tsl is required for Trk cleavage. Surprisingly, we find that Trk cleavage can take place in the absence of Tsl. One explanation for these data is that most Trk cleavage events are independent of Tsl, and that a small amount of Tsl-dependent changes in Trk cleavage occurring only at the embryo poles cannot be detected. Alternatively, we argue that our data favour a model where Tsl functions post proteolytic processing of Trk to control localized terminal patterning. Trk is cleaved multiple times To investigate Trk activation, we set out to ascertain whether Trk cleavage is required for terminal patterning. We were unable to generate satisfactory antibodies for Trk; hence, we generated transgenic flies carrying various N- and C-terminally tagged forms of Trk. To ensure further studies were performed on a functional Trk protein, we first determined which of the tagged proteins could successfully rescue trk -null mutants. Since available stocks carrying trk- mutant alleles are likely hypomorphic and/or have additional genetic mutations, ends-out gene replacement was used to generate a trk- null mutant allele ( trk Δ ) in which the entire coding region is removed ( Fig. 1 ). trk Δ homozygotes are viable but females are sterile, laying embryos that fail to specify terminal cell fate ( Fig. 1 ). 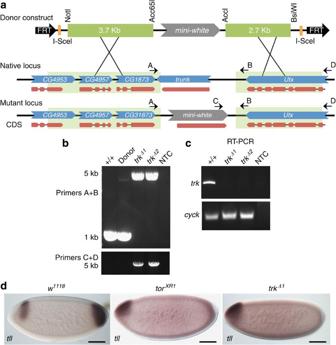Figure 1: Generation of atrk-null mutant via ends-out gene targeting. (a) Targeting scheme for the removal of thetrkcoding sequence using ends-out gene replacement. The donor construct was generated by cloning 2.7 kb of upstream and 3.7 kb of downstream flanking sequence. (b) Verification oftrk-targeted events. Primers A and B span the targeted region and amplify 5 kb whentrkhas been replaced by the white gene from pw25 (1 kb amplicon results from untargeted locus). Primers C and D amplify 5 kb only when targeting events have occurred. (c) RT–PCR confirms lack oftrktranscripts in twotrk-null mutant lines (400 bp amplicon is present in wild-type control, thecycK-positive control amplicon is 145 bp, NTC, no template control). (d) RNAin situhybridization of early embryos with a probe totailless (tll), a zygotic gene that is transcribed in response to Tor signalling. Embryos laid bytrkΔfemales display defectivetllexpression identical to that observed in embryos maternally lackingtor (torXR1), indicating a failure to specify terminal fate. Scale bars, 100 μm. Anterior is positioned to the left. Figure 1: Generation of a trk- null mutant via ends-out gene targeting. ( a ) Targeting scheme for the removal of the trk coding sequence using ends-out gene replacement. The donor construct was generated by cloning 2.7 kb of upstream and 3.7 kb of downstream flanking sequence. ( b ) Verification of trk -targeted events. Primers A and B span the targeted region and amplify 5 kb when trk has been replaced by the white gene from pw25 (1 kb amplicon results from untargeted locus). Primers C and D amplify 5 kb only when targeting events have occurred. ( c ) RT–PCR confirms lack of trk transcripts in two trk- null mutant lines (400 bp amplicon is present in wild-type control, the cycK- positive control amplicon is 145 bp, NTC, no template control). ( d ) RNA in situ hybridization of early embryos with a probe to tailless (tll) , a zygotic gene that is transcribed in response to Tor signalling. Embryos laid by trk Δ females display defective tll expression identical to that observed in embryos maternally lacking tor (tor XR1 ), indicating a failure to specify terminal fate. Scale bars, 100 μm. Anterior is positioned to the left. Full size image Several combinations of large (fluorescent protein) and small (epitope) tags revealed the N terminus of Trk to be insensitive to tagging ( Fig. 2a ). While Trk function was lost upon C-terminal fusion with GFP, addition of smaller epitopes to the C-terminus had no functional consequences ( Fig. 2 ). Expression of one functional C-terminally tagged Trk protein, HA:Trk:Myc, was detectable in embryo samples by immunoblotting for the Myc tag (35 kDa, Fig. 3a ). Importantly, concentration of the fusion protein in embryo extracts via immunoprecipitation revealed the presence of at least six C-terminal Trk fragments ranging from 10–35 kDa ( Fig. 3b ). This is consistent with the idea that Trk may undergo several cleavage events. We note that although this construct has both N-terminal hemagglutinin (HA) and C-terminal Myc tags, only the full-length fusion protein was detected with anti-HA; no smaller N-terminal Trk fragments could be detected after immunoprecipitation ( Fig. 3c ). As we have only been able to detect full-length N-terminally tagged protein, it is possible that the N-terminal region, once removed, is rapidly degraded. 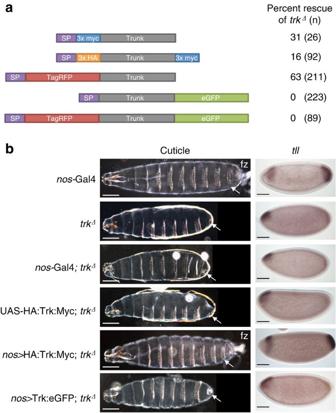Figure 2: Rescue of thetrkΔterminal phenotype by expression of a tagged form of Trk. (a) Schematic representation of tagged Trk proteins that were tested for their ability to rescue thetrkΔ-mutant phenotype. The N-terminal signal sequence of Trk (purple box, SP) was used in all cases. The relative ability of the individual fusion proteins to rescue thetrkΔ-mutant phenotype is indicated. (b) The wild-type control (nos-Gal4) first-instar larval cuticle shows the presence of normal terminal structures, including abdominal segments posterior to A7 (arrowed) and the filzkorper (fz) and normaltailless (tll)expression. ThetrkΔcuticle lacks abdominal segments posterior to A7 and filzkorper, and shows an alteredtllexpression pattern with complete loss at the posterior (typical of a terminal-class mutant). We found that for individual embryos, maternal expression of Trk withnos-Gal4 gave either complete rescue (wild-type phenotype) or no rescue at all (trkΔphenotype), representative examples of each are shown (HA:Trk:Myc rescues, Trk:eGFP does not). Scale bars, 100 μm. Anterior is to the left and maternal genotypes are as indicated. For each experiment at least two independent transgenic Trk lines were tested. Figure 2: Rescue of the trk Δ terminal phenotype by expression of a tagged form of Trk. ( a ) Schematic representation of tagged Trk proteins that were tested for their ability to rescue the trk Δ -mutant phenotype. The N-terminal signal sequence of Trk (purple box, SP) was used in all cases. The relative ability of the individual fusion proteins to rescue the trk Δ -mutant phenotype is indicated. ( b ) The wild-type control ( nos -Gal4) first-instar larval cuticle shows the presence of normal terminal structures, including abdominal segments posterior to A7 (arrowed) and the filzkorper (fz) and normal tailless (tll) expression. The trk Δ cuticle lacks abdominal segments posterior to A7 and filzkorper, and shows an altered tll expression pattern with complete loss at the posterior (typical of a terminal-class mutant). We found that for individual embryos, maternal expression of Trk with nos- Gal4 gave either complete rescue (wild-type phenotype) or no rescue at all ( trk Δ phenotype), representative examples of each are shown (HA:Trk:Myc rescues, Trk:eGFP does not). Scale bars, 100 μm. Anterior is to the left and maternal genotypes are as indicated. For each experiment at least two independent transgenic Trk lines were tested. 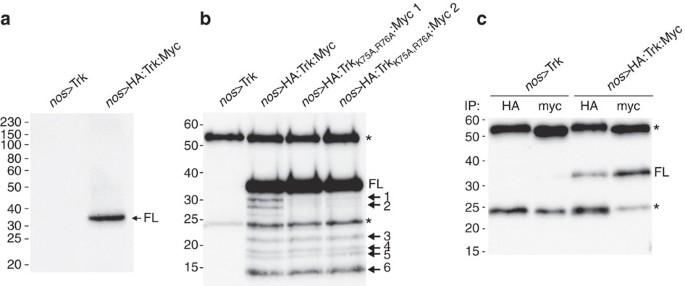Figure 3: Trk is cleaved multiple times. (a) Immunoblot without prior immunoprecipitation of protein extracted from embryos expressing HA:Trk:Myc. Only full-length Trk (FL) is detected using anti-Myc. (b) Immunoblot of protein extracts immunoprecipitated (using anti-Myc) from embryos expressing Trk constructs and blotted with anti-Myc. HA:Trk:Myc extracts contain a predominant Trk species (FL=full length) and at least six C-terminal Trk fragments (arrows) not observed in untagged Trk extracts (nos>Trk). Two independent TrkK75A,R76Amutants lack fragments 1 and 2. (c) Immunoblot of protein extracts immunoprecipitated (using anti-Myc or anti-HA) from embryos expressing HA:Trk:Myc and blotted with anti-HA. Note that full-length (FL) Trk protein immunoprecipitated with anti-Myc can be detected with anti-HA. No additional N-terminal Trk fragments are observed in extracts immunoprecipitated with anti-HA. * indicates immunoglobulin bands. Images are representative of at least two replicate immunoblots. Full size image Figure 3: Trk is cleaved multiple times. ( a ) Immunoblot without prior immunoprecipitation of protein extracted from embryos expressing HA:Trk:Myc. Only full-length Trk (FL) is detected using anti-Myc. ( b ) Immunoblot of protein extracts immunoprecipitated (using anti-Myc) from embryos expressing Trk constructs and blotted with anti-Myc. HA:Trk:Myc extracts contain a predominant Trk species (FL=full length) and at least six C-terminal Trk fragments (arrows) not observed in untagged Trk extracts ( nos >Trk). Two independent Trk K75A,R76A mutants lack fragments 1 and 2. ( c ) Immunoblot of protein extracts immunoprecipitated (using anti-Myc or anti-HA) from embryos expressing HA:Trk:Myc and blotted with anti-HA. Note that full-length (FL) Trk protein immunoprecipitated with anti-Myc can be detected with anti-HA. No additional N-terminal Trk fragments are observed in extracts immunoprecipitated with anti-HA. * indicates immunoglobulin bands. Images are representative of at least two replicate immunoblots. Full size image Trk cleavage is required for terminal patterning Given these data, we were then in a position to investigate whether Trk cleavage is required for its function. Previously, Casanova et al. [5] predicted a possible cleavage site at R76-S77 via local sequence similarity to a cleavage sequence present in complement C3. We further noted that a dibasic motif (K75 and R76 in D. melanogaster Trk) is conserved across Trk proteins from different Drosophila species, as well as in other insect Trk proteins, consistent with a recognition sequence for a target protease ( Fig. 4a ). Because Trk shares significant sequence similarity and domain architecture to the mammalian growth factor Noggin (ref. 1 and Fig. 4b ), we analysed the Trk sequence with respect to the X-ray crystal structure of Noggin [2] . This revealed that K75-R76 likely maps to a mobile (disordered in electron density) exposed loop that could be accessible by a target protease ( Fig. 4c ). To test this, we performed an in vivo alanine scan of Trk across residues H71-P82, using the rescue of terminal patterning in trk Δ mutants as an assay for function ( Fig. 4d ). Both the K75A and R76A mutations abolished Trk function ( Fig. 4d,e ). In contrast, Trk proteins containing mutations N- or C-terminal of these two amino-acid positions retained function ( Fig. 4d ). 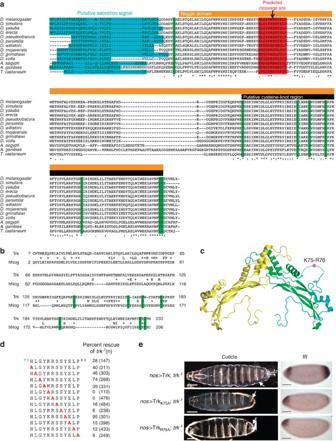Figure 4: Cleavage of Trk at K75-R76 is required for terminal patterning. (a) Alignment of insect Trk-like proteins annotated with putative secretion signal (cyan), conserved cysteines (green), predicted cleavage site (arrowed) and surrounding sequence (red). Orange bar indicates a region of significant sequence conservation with the Noggin domain (EXPECT 2.97 × 10−6forD. melanogaster, pfam05806). Black bar denotes the putative cysteine-knot region. (b) Alignment from PSI-BLAST search showing the pairwise match between human Noggin andD. melanogasterTrk (EXPECT score 6 × 10−49, where scores below 1 × 10−6are considered significant37). Conserved cysteine residues that form the 3D cysteine knot structure in Noggin are highlighted in green. (c) X-ray crystal structure of the Noggin dimer2(pdb identifier 1M4U) with constituent monomers in green and yellow. The region equivalent to the Trk N-terminus1(mapped using PSI-BLAST alignments) is in cyan on one monomer. K75-R76 in Trk maps to an exposed loop in the N-terminus that is mobile and not visible in electron density (dashed line). Image produced using PyMOL. (d) Alanine scan of putative Trk cleavage site. Twelve constructs, each containing a single-alanine substitution, were tested for rescue of thetrkΔphenotype (level of rescue is indicated). (e) Rescue was not observed for TrkK75Aand TrkR76Amutations; anterior is to the left, maternal genotypes indicated. Scale bars, 100 μm. For each experiment at least two independent transgenic Trk lines were tested. Figure 4: Cleavage of Trk at K75-R76 is required for terminal patterning. ( a ) Alignment of insect Trk-like proteins annotated with putative secretion signal (cyan), conserved cysteines (green), predicted cleavage site (arrowed) and surrounding sequence (red). Orange bar indicates a region of significant sequence conservation with the Noggin domain (EXPECT 2.97 × 10 −6 for D. melanogaster , pfam05806). Black bar denotes the putative cysteine-knot region. ( b ) Alignment from PSI-BLAST search showing the pairwise match between human Noggin and D. melanogaster Trk (EXPECT score 6 × 10 −49 , where scores below 1 × 10 −6 are considered significant [37] ). Conserved cysteine residues that form the 3D cysteine knot structure in Noggin are highlighted in green. ( c ) X-ray crystal structure of the Noggin dimer [2] (pdb identifier 1M4U) with constituent monomers in green and yellow. The region equivalent to the Trk N-terminus [1] (mapped using PSI-BLAST alignments) is in cyan on one monomer. K75-R76 in Trk maps to an exposed loop in the N-terminus that is mobile and not visible in electron density (dashed line). Image produced using PyMOL. ( d ) Alanine scan of putative Trk cleavage site. Twelve constructs, each containing a single-alanine substitution, were tested for rescue of the trk Δ phenotype (level of rescue is indicated). ( e ) Rescue was not observed for Trk K75A and Trk R76A mutations; anterior is to the left, maternal genotypes indicated. Scale bars, 100 μm. For each experiment at least two independent transgenic Trk lines were tested. Full size image Having demonstrated the functional importance of the K75-R76 sequence, we investigated whether the K75A and R76A mutations impacted on Trk cleavage. Strikingly, the Trk K75A,R76A mutation resulted in the loss of two C-terminal Trk fragments ( Fig. 3b ), thus identifying K75 and R76 as key determinants of specificity for Trk cleavage. Further, together with our earlier findings, these data demonstrate that abolishing a Trk cleavage event is directly associated with loss of Trk function. Importantly, for the first time, these data also demonstrate an ability to detect changes in Trk cleavage patterns in vivo . Tsl does not influence the observed Trk cleavage pattern Finally, we sought to test the current model that Tsl is required for Trk cleavage. This was achieved by expressing the HA:Trk:Myc construct in a tsl -null mutant background. Unexpectedly, we saw no difference in the Trk cleavage pattern in the absence of Tsl ( Fig. 5a ). Given that Tor signalling only occurs at the embryo poles, there may be a small amount of Tsl-dependent Trk cleavage product that is below the detection level of our assay. To address this, we ectopically produced Tsl from all ovarian follicle cells using c355 -Gal4 (ref. 15) [15] while also producing tagged Trk from the germline. Unrestricted expression of Tsl results in ubiquitous Tor activation and causes the spliced cuticle phenotype—an expansion of the terminal regions at the expense of central segments (ref. 10 and Fig. 5b ). We reasoned that under this scenario, the abundance of a Tsl-dependent Trk cleavage product should be greatly increased. However, we did not observe any additional Trk cleavage products in these embryos ( Fig. 5c ). 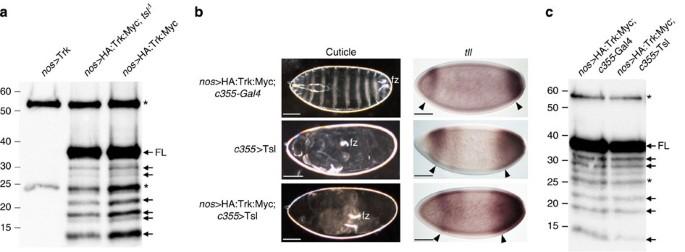Figure 5: Trk cleavage occurs independently of Tsl function. (a) Protein was extracted and immunopreciptated (anti-Myc) from embryos expressing HA:Trk:Myc. Note that all observed C-terminal Trk fragments (arrows) are also present in the absence of Tsl (tslΔ). (b) Representative cuticles andtll in situhybridizations of embryos laid by mothers of the genotype indicated. Ectopic expression of Tsl usingc355-Gal4 results in an un-segmented embryo with a centrally positioned filzkorper (fz) and greatly expandedtlldomain (arrowed). When HA:Trk:Myc is overexpressed from the germline in this background, the phenotype is unchanged. Anterior is to the left. Scale bars, 100 μm. (c) No additional Trk-cleavage products are observed when Tsl is ectopically expressed. * indicates immunoglobulin bands. FL=full length. Images are representative of at least two repeat experiments. Figure 5: Trk cleavage occurs independently of Tsl function. ( a ) Protein was extracted and immunopreciptated (anti-Myc) from embryos expressing HA:Trk:Myc. Note that all observed C-terminal Trk fragments (arrows) are also present in the absence of Tsl ( tsl Δ ). ( b ) Representative cuticles and tll in situ hybridizations of embryos laid by mothers of the genotype indicated. Ectopic expression of Tsl using c355- Gal4 results in an un-segmented embryo with a centrally positioned filzkorper (fz) and greatly expanded tll domain (arrowed). When HA:Trk:Myc is overexpressed from the germline in this background, the phenotype is unchanged. Anterior is to the left. Scale bars, 100 μm. ( c ) No additional Trk-cleavage products are observed when Tsl is ectopically expressed. * indicates immunoglobulin bands. FL=full length. Images are representative of at least two repeat experiments. Full size image Taken together, our data strongly support the idea that Trk must be cleaved in order to bind and activate the Tor receptor. While the Trk cleavage products that we detect are produced independently of Tsl, we cannot completely eliminate the possibility that the localized influence of Tsl on Trk cleavage events is extremely subtle, and lies beyond what we are able to detect. Alternatively, we argue that a simpler explanation for our data is that Tsl acts in terminal patterning after Trk cleavage. In this latter scenario, if Trk does not require Tsl for proteolytic activation, then how could localized Trk/Tor signalling be achieved? One possibility is that activated Trk requires Tsl for binding to Tor. However, this seems unlikely as Sprenger and Nüsslein-Volhard [11] elegantly demonstrated that the Tor ligand can diffuse and activate Tor that is artificially localized to only the middle of the embryo. This cannot require direct participation by Tsl, as Tsl is localized to the embryo poles via its interaction with the vitelline membrane and is not present elsewhere in the embryo [16] . Further, we have not been able to detect direct interactions between Trk/Tor/Tsl in co-immunoprecipitation experiments. We thus propose an alternative hypothesis for the events that surround localized Trk/Tor signalling. Tsl shares no sequence similarity to any known protease family, and instead is a member of the cholesterol-dependent cytolysin (CDC)/MACPF superfamily [17] , [18] . The primary characterized function of this protein superfamily is in pore formation and/or membrane disruption [18] , [19] , [20] , [21] , [22] ; however, it has not been considered how such a role might relate to localized Trk/Tor signalling. In this regard, it is notable that a general response to membrane damage (including pore-induced lesions) involves local stimulation of both endocytosis and exocytosis as part of the membrane repair response [23] , [24] , [25] , [26] , [27] . For example, it has been shown that the pore-forming toxin Streptolysin O (a member of the CDC/MACPF superfamily) induces exocytosis of lysosomes and the release of enzymes required for membrane repair [28] , [29] . This may represent an ancient defensive response to pathogen attack [25] , [30] , [31] , [32] . Accordingly, given a known role for CDC/MACPF proteins in exocytosis, we suggest that the trafficking machinery required for active Trk secretion may be Tsl dependent. Drosophila stocks The following stocks were used: hs-FLP hs-I-SceI (BL6935), ey - FLP (BL5580), w 1118 (BL5905), Gal4::VP16-nos.UTR (BL7293), c355-Gal4 (BL3750), UAS- tsl (ref. 7 ), tsl Δ , a null mutant of torso-like (ref. 7 ) and tor XR1 , a small deficiency uncovering the torso locus [8] (gift from Dr. Jordi Casanova). Generation of trk -null mutants and transgenic lines The trk- null mutant was generated using ends-out gene replacement [33] . First, the donor plasmid pW25-trk was built by cloning 2.7 Kbp of upstream (F- 5′-AGCAGGCGCGCCTTCAGTGTCATTGCGAAAGATT-3′, R-5′-TACCCGTACGCAGTGGGCAATCAACTAAATCA-3′) and 3.7 Kbp of downstream (F-5′-AGCAGCGGCCGCGAGAAGGGCAGACTGCAAAC-3′, R-5′-TACCGGTACCTTGATTTTGATCACCGCAGA-3′) sequence flanking the trk coding region into the appropriate sites in the ends-out transformation vector pW25. For pW25- trk and other Trk constructs, transgenics were generated by injection into w 1118 embryos (BestGene) using standard protocols [34] . The donor targeting element was mobilized by crossing to hs-FLP, hs-I-SceI and applying a heat shock for 80 min at 37 °C daily for days 3–5 of development. Mosaic and white-eyed virgins were crossed to ey -FLP and stable lines were established from w+ progeny (~1/6 vials yielded a w+ individual). Lines were characterized for targeting events via PCR (A-5′-CCAGCTTGGTGGTTAAGAGC-3′, B-5′-AGCCCACTTGAGTAGCGAAA-3′, C-5′-AGACAACGGTGAGTGGTTCC-3′, D-5′-CCAAGACAGGTCACAAAGCA-3′). Of the 14 w+ lines we generated, two had undergone gene replacement. trk transcriptional activity was assessed in the mutants by RT–PCR from ovary derived cDNA using primers specific for trk (F-5′-TTCTATGCGGACAGTGATGC-3′, R-5′-CCAAATCCAGAGCTGCGTA-3′) and a control gene CyclinK (F-5′-GAGCATCCTTACACCTTTCTCCT-3′, R-5′-TAATCTCCGGCTCCCACTG-3′). Wild-type, tagged and mutant Trk constructs, were synthesized, mutated (where necessary) and cloned (Genscript) into pUASP [35] . The N-terminal tags, 3xMyc, 3xHA and TagRFP, were spliced into the Trk sequence between residues D34-Y35 and flanked with a short linker peptide (SAGSAS). C-terminal tags (3 × Myc, eGFP) were fused directly to the last residue encoded by the trk sequence. For all transgenes, several independent transgenic lines were established and tested. RNA in situ hybridizations T7 RNA polymerase (Roche) was used to transcribe a 980 bp fragment of tll (F-5′-AGTGCTTTGAGGTCGGAATG-3′, R-5′-TTGAGACCTTGTGCATCAGC-3′) that had been cloned into pGEM-T easy (Promega) to produce a DIG-labelled antisense RNA probe. In situ hybridization on whole-mount embryos was performed using standard protocols [36] before imaging with differential interference contrast optics on a Leica DM LB compound microscope. Cuticle preparations Adults were allowed to lay on media containing apple juice supplemented with yeast paste for 24 h before being removed. Embryos were developed for further 24 h before dechorionation in 50% vol/vol bleach and mounting on slides in a mixture of 1:1 Hoyer’s solution: lactic acid. Slides were incubated overnight at 65 °C and imaged using dark field optics (Leica). Protein extraction and immunoprecipitation Approximately 500 μl volume of 0–6 h-old embryos were homogenized in lysis buffer (50 mM Tris–HCl (pH 7.5), 150 mM NaCl, 2.5 mM EDTA, 0.2% Triton X, 5% glycerol, complete EDTA-free protease inhibitor cocktail (Roche)) and spun at 500 g for 5 mins at 4 °C. The supernatants obtained were made up to 1 ml with lysis buffer and incubated with 2 μl anti-Myc (Cell Signalling, 9B11) or 6 μl anti-HA (Roche, 12CA5) overnight at 4 °C. Protein A sepharose beads (100 μl, GE Healthcare; CL-4B) in lysis buffer were added and extracts were incubated for another 4 h. The beads were collected by centrifugation, washed four times with lysis buffer and bound protein was removed via boiling in 40 μl sample buffer containing 6 M urea. Equal amounts of protein were separated by SDS–PAGE (12%) and transferred onto Immobilon-P membrane (Millipore). Membranes were probed with 1:1,000 anti-Myc (Cell Signalling; 9B11) or 1:1,000 anti-HA (Roche, 12CA5), washed and incubated with HRP-conjugated secondary antibody (1:10,000, Southern Biotech). Immunoblots were developed using ECL (GE healthcare) and imaged using a chemiluminescence detector (Vilber Lourmat). Bioinformatics The alignment of Noggin and Trunk was produced using the results of PSI-BLAST searches [37] using a significance cut-off of 1 × 10 −6 in the first 20 interactions [38] . The structure of Noggin was obtained from the pdb (1M4U, chain A), and Figure 4c produced using PYMOL (Schrödinger, LLC.) Trunk-like protein sequences from various insect species were taken from OrthoDB [39] and aligned using Clustal Omega [40] . The alignment was manually adjusted to correct for obvious misalignments and to reflect structural insights derived from 1M4U and other cysteine-knot proteins. SignalP 4.0 (ref. 41) [41] was used to annotate putative secretion signals and the Conserved Domains Database [42] for determining regions of Trk bearing the Noggin domain. How to cite this article : Henstridge, M. A. et al. Trunk cleavage is essential for Drosophila terminal patterning and can occur independently of Torso-like. Nat. Commun. 5:3419 doi: 10.1038/ncomms4419 (2014).